Metal-templated chiral Brønsted base organocatalysis Inert octahedral chiral-at-metal complexes are an emerging class of asymmetric catalysts that exploit the globular, rigid nature and stereochemical options of octahedral compounds. While the central transition metal serves as a structural anchorpoint and provides metal centrochirality, catalysis is mediated through the organic ligand sphere, thereby merging the branches of transition metal catalysis and organocatalysis. Here we report the development of inert octahedral 3-aminopyrazolato iridium(III) complexes as novel chiral Brønsted base catalysts and demonstrate their merit with applications to highly effective asymmetric sulfa-Michael and aza-Henry reactions, permitting catalyst loadings down to 0.02 and 0.25 mol%, respectively. The observed high stereocontrol can be rationalized by a bifunctional mode of action in which the iridium catalyst, after the initial proton transfer, controls a ternary complex through defined hydrogen bonding interactions. This work reveals the potential of octahedral metal complexes as chiral scaffolds for the design of high-performance asymmetric catalysts. The demand for ever more sophisticated asymmetric catalysts in chemistry is driven by industrial applications of optical active intermediates and products. Dual activation by multifunctional catalysts has unfolded as a powerful generic concept for the design of high-performance asymmetric metal-based catalysts [1] , [2] , [3] , [4] , [5] and asymmetric organocatalysts [6] , [7] , [8] , [9] , [10] , [11] , [12] , [13] . For prototypical bimolecular reactions, such catalysts simultaneously interact through two or more functional groups (bifunctional or multifunctional catalysis) with both reaction partners (dual activation catalysis), thereby achieving a synergistic electronic activation of both substrates and their positioning in close proximity with the required orientation so that the reaction can proceed with high-rate acceleration and a defined transfer of stereochemical information from the catalyst to the product, very much in analogy to enzyme catalysis. However, the design of truly high-performance multifunctional catalysts poses significant practical challenges as cooperativity of the involved functional groups, and hence their proper positioning and orientation within the chiral catalyst scaffold, is a prerequisite for gaining a maximum catalytic activity and high asymmetric induction. Structurally diverse chemical scaffolds may therefore greatly contribute to multifunctional dual activation catalysis so that the theoretically possible rate acceleration and asymmetric induction can be reached. Proton transfer is one of the most prevalent elementary steps for activating substrates towards chemical reactions [14] . The advent of asymmetric organocatalysis over the last decade has consequently witnessed large activities in the development of chiral Brønsted acid and base catalysts [15] , [16] , [17] , [18] , [19] . Interestingly, with respect to chiral Brønsted base catalysis, although such chiral Brønsted bases have been reported as powerful catalysts for a range of asymmetric transformations, the vast majority of such catalysts is based on a limited number of basic functional groups—mainly tertiary amines, amidines and guanidines, and more recently also cyclopropenimines [20] and iminophosphoranes [21] ( Fig. 1a )—and just a few underlying substance classes, particularly cinchona alkaloids, bifunctional thiourea and 1,1′-binaphthyl derivatives ( Fig. 1b ) (refs 17 , 18 , 19 ). Clearly, novel chiral Brønsted bases built on yet unexplored platforms are desired to provide new opportunities for basicity tuning and/or bi- or multifunctional catalyst design. 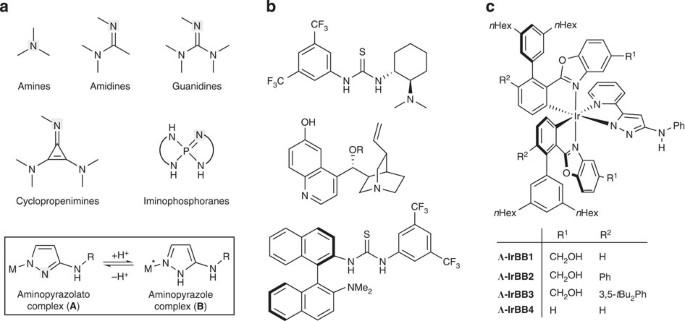Figure 1: Brønsted base catalysts. (a) Typical nitrogen bases used for asymmetric Brønsted base catalysis compared with chiral 3-aminopyrazolato metal complexes used in this study. (b) Examples of bifunctional chiral Brønsted base catalysts. (c) Design of chiral-at-metal octahedral IrIIIcomplexes as bifunctional, asymmetric Brønsted base catalysts. SeeSupplementary Methodsfor the synthesis of the non-racemic chiral iridium complexes Λ-IrBB1-4. Figure 1: Brønsted base catalysts. ( a ) Typical nitrogen bases used for asymmetric Brønsted base catalysis compared with chiral 3-aminopyrazolato metal complexes used in this study. ( b ) Examples of bifunctional chiral Brønsted base catalysts. ( c ) Design of chiral-at-metal octahedral Ir III complexes as bifunctional, asymmetric Brønsted base catalysts. See Supplementary Methods for the synthesis of the non-racemic chiral iridium complexes Λ- IrBB1 - 4 . Full size image We recently introduced octahedral chiral-at-metal [22] , [23] , [24] , [25] , [26] , [27] , [28] , [29] , [30] , [31] , [32] , [33] , [34] , [35] iridium(III) complexes as inert templates for the design of low-loading asymmetric hydrogen bonding catalysts [36] , [37] . Octahedral stereocenter [38] , [39] , [40] permit the straightforward generation of compounds with high shape and stereochemical complexity and should therefore be highly suitable as structural templates for multifunctional catalysts. Octahedral stereocenter furthermore simplify the design of defined globular and rigid structures as molecular geometries are basically constructed from a common centre with steric crowding and chelating ligands limiting the degree of conformational flexibility [41] . This limited flexibility is not only advantageous for entropic reasons but also facilitates the intuitive and rational catalyst optimization. Herein, we now demonstrate how octahedral chiral-at-metal complexes can serve as effective templates for the design of novel chiral Brønsted bases, namely inert chiral-at-metal 3-aminopyrazolato iridium(III) complexes ( Fig. 1c ), which serve as chiral Brønsted base/H-bonding dual activation asymmetric catalysts. Catalysis with these complexes is exclusively conducted through the tailored arrangement of functional groups in the metal-coordinated organic ligands, whereas the metal itself is not involved in any direct interaction and its centrochirality serves as the sole source for the asymmetric induction. We demonstrate the versatility of this class of chiral iridium-based Brønsted base catalysts as high-performance catalysts for the asymmetric sulfa-Michael (down to 0.02 mol% catalyst loading) and aza-Henry (down to 0.25 mol% catalyst loading) reaction. Metal-templated catalyst design Recently, we reported iridium-coordinated pyrazole complexes as asymmetric H-bonding catalysts [36] , [37] . We hypothesized that the corresponding deprotonated pyrazolato complexes might serve as chiral Brønsted bases with an amino group in the 3-position of the coordinated pyrazolato ligand [42] , [43] , [44] ( A in Fig. 1a ) raising the basicity and serving as part of a double hydrogen acceptor site on protonation to the 3-aminopyrazole complex ( B in Fig. 1a ). Accordingly, we started our study with the substitutionally and configurationally inert bis-cyclometalated iridium(III) complex [45] Λ- IrBB1 containing a basic 3-( N -phenylamino)-5-(pyridin-2-yl)pyrazolato bidentate ligand for activating a nucleophile on deprotonation, hydroxymethyl groups at the cyclometalated ligands as additional hydrogen bond donors for activating incoming electrophiles, and hexyl groups for improving the solubility in aprotic solvents ( Fig. 1c ). A crystal structure of a derivative of Λ- IrBB1 is shown in Fig. 2 and confirms the proposed molecular structure having a deprotonated pyrazolato ligand coordinated to the iridium ( A in Fig. 1a ). The exocyclic amino group is somewhat rotated out of planarity, which might be at least in parts due to crystal packing effects. 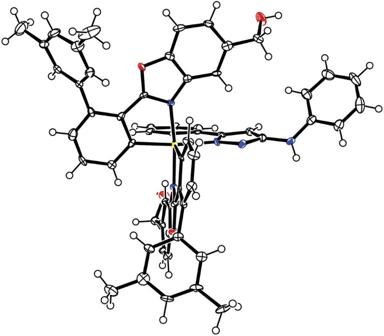Figure 2: Crystal structure of a derivative of Λ-IrBB1 (Λ-IrBB1'). Then-hexyl groups of Λ-IrBB1are replaced by methyl groups for improved crystallization behaviour. ORTEP drawing with 50% probability thermal ellipsoids including calculated positions of hydrogen atoms. Solvent is omitted for clarity. Figure 2: Crystal structure of a derivative of Λ-IrBB1 (Λ-IrBB1'). The n -hexyl groups of Λ- IrBB1 are replaced by methyl groups for improved crystallization behaviour. ORTEP drawing with 50% probability thermal ellipsoids including calculated positions of hydrogen atoms. Solvent is omitted for clarity. Full size image Asymmetric sulfa-Michael additions When applied to the sulfa-Michael addition [46] , [47] , [48] , [49] , [50] , [51] , [52] , [53] , we were pleased to find that the reaction of N -pyrazolylcrotonate ( 1a ) with p -methylbenzenethiol ( 2a ) provided after 12 h at −78 °C the addition product ( R )- 3a in 96% yield and 97% ee just using 0.05 mol% Λ- IrBB1 ( Table 1 , entry 1), whereas, as expected, the previously designed H-bonding iridium catalysts [36] , [37] did not catalyse this reaction ( Supplementary Table 1 ). Even with a catalyst loading of merely 0.02 mol% Λ- IrBB1 , ( R )- 3a was obtained in unchanged high yield (96%) and with high enantioselectivity (96%) (entry 2), reflecting a turnover number of 4,800. The reaction works with more bulky (entries 3 and 7), electron rich (entries 4 and 5), and electron deficient (entry 6) arenethiols, the aliphatic thiol BnSH (entry 8), as well as N -pyrazolyl-( E )-2-hexenoate ( 1b ) (entry 9) and the CF 3 -substituted alkene N -pyrazolyl-4-trifluorocrotonate ( 1c ) (entry 10). Table 1 Asymmetric sulfa-Michael reaction catalysed by an inert chiral-at-metal Ir III catalyst*. Full size table Asymmetric aza-Henry reactions We decided to next investigate the asymmetric formation of a C–C bond and selected the aza-Henry (nitro-Mannich) reaction [54] . Encouragingly, the reaction between (nitromethyl)benzene ( 4a ) and N -Boc-Schiff base 5a (refs 55 , 56 , 57 ), a reaction that cannot be catalysed by our previously developed H-bonding iridium complexes ( Supplementary Table 2 ) [36] , [37] , afforded in the presence of Λ- IrBB1 the C–C bond formation product (1 R ,2 S )- 6a under the implementation of two stereocenters with 92% ee and 122:1 dr , albeit requiring a high catalyst loading of 10 mol% ( Table 2 , entry 1). Reducing the catalyst loading to 1 mol% diminished the enantiomeric excess to just 71% (entry 2). However, when introducing a phenyl group next to the 3,5-( n Hex) 2 Ph moiety (Λ- IrBB2 ), (1 R ,2 S )- 6a was formed with 86% ee employing only 1 mol% catalyst loading (entry 3). Increasing the steric demand further by introducing additional t Bu-groups (Λ- IrBB3 ) improved the enantioselectivity to 94% ee at 1 mol% catalyst loading at −20 °C (entry 4). A decreased temperature of −45 °C even allowed to reduce the catalyst loading further (0.25 mol%), while maintaining a high ee value of 94% (entry 5). 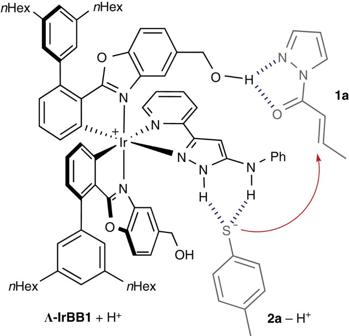Figure 3: Mechanism of sulfa-Michael reaction. Proposed ternary complex for the reaction1a+2a→(R)-3acatalysed by Λ-IrBB1. It is noteworthy that theR-configuration of the sulfa-Michael addition products render a mechanism unlikely in which instead the α,β-unsaturatedN-acyl pyrazole hydrogen bonds with the aminopyrazole ligand. With respect to substrate scope, as shown in Table 3 , the reaction of different arylnitromethanes ( 4a – f ) with a variety of substituted N -Boc-Schiff bases ( 5a – e ) provided the desired β-nitrocarbamates all with high enantio- (91-98% ee ) and diastereoselectivities (22:1 to >300:1 dr ) in the presence of just 0.25 mol% Λ- IrBB3 (entries 1–10). Furthermore, the reaction is also amenable to (phenylthio)nitromethane ( 4g ), which provided the aza-Henry product with 90% ee and 13:1 dr (entry 11). It is also noteworthy that the catalyst can be recycled and used again without any loss of performance ( Supplementary Methods ). Table 2 Development of inert chiral-at-metal Ir III catalysts for the asymmetric aza-Henry reaction*. Full size table Table 3 Scope of the asymmetric aza-Henry reaction catalysed by Λ-IrBB3*. Full size table Mechanistically, for the sulfa-Michael addition, we propose that that after an initial activating proton transfer from the acidic thiol (p K a ~10 in dimethylsulphoxide for PhSH) [58] to the iridium Brønsted base (p K a ~16 of protonated Λ- IrBB1 in MeCN, Supplementary Methods ), the formed ion pair out of thiolate and cationic iridium complex aggregates through a double hydrogen bond with the aminopyrazole ligand. Related two-point hydrogen bonds of thiourea to single atoms of organic or inorganic anions are well established [11] . It is then plausible that the α,β-unsaturated N -acyl pyrazole electrophile undergoes a three-centre hydrogen bond with the hydroxymethyl substituent of the benzoxazole moiety, thereby arranging a ternary complex through hydrogen bonding and electrostatic attraction that allows the Michael addition to proceed with high-rate acceleration and high asymmetric induction ( Fig. 3 ). 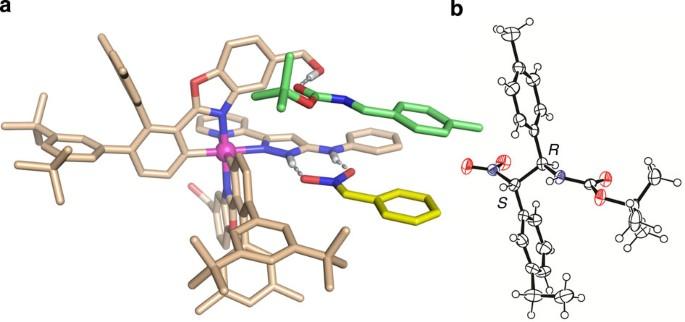Figure 4: Mechanism of the aza-Henry reaction. (a) Proposed hydrogen-bonded ternary complex composed of a simpified derivative of iridium catalyst Λ-IrBB3(wheat), deprotonated (nitromethyl)benzene (yellow) andN-Boc-Schiff base5a(green) leading to the transitions state for the formation of (1R,2S)-6a. The ternary complex was built with the molecular modelling software Scigress (Fujitsu) and represented with the PyMOL Molecular Graphics System, Version 1.3 Schrödinger, LLC. (b) ORTEP representation with 50% probability thermal ellipsoids of a crystal structure of (1R,2S)-6g. Solvent is omitted for clarity. The formation of such a ternary complex held together by a network of hydrogen bonds is supported by control experiments in which we replaced the strong hydrogen bond accepting pyrazolyl [59] group of substrate 1a with an ethoxy group ( Supplementary Table 3 ) or deleted the hydroxymethyl groups of Λ- IrBB1 ( Supplementary Table 4 ). In both instances, only sluggish catalysis was observed. Figure 3: Mechanism of sulfa-Michael reaction. Proposed ternary complex for the reaction 1a + 2a →( R )- 3a catalysed by Λ- IrBB1 . It is noteworthy that the R -configuration of the sulfa-Michael addition products render a mechanism unlikely in which instead the α,β-unsaturated N -acyl pyrazole hydrogen bonds with the aminopyrazole ligand. Full size image Regarding the mechanism of the aza-Henry reaction, the observed high stereocontrol can be rationalized by a bifunctional mode of action in which the iridium catalyst—after the initial proton transfer between catalyst and nitro substrate (p K a ~12 in dimethylsulphoxide) [60] —controls a ternary complex with the intermediate nitronate anion and the N -Boc-Schiff base through defined hydrogen bonds as displayed in Fig. 4a . This mode of action is consistent with the observed absolute 1 R ,2 S -configuration of the formed β-nitrocarbamates ( Fig. 4b ) and is further supported by results obtained with the catalyst Λ- IrBB4 devoid of the hydroxymethyl groups. As shown in Table 2 (entry 6), the reaction 4a + 5a →(1 R ,2 S )- 6a catalysed by 3 mol% Λ- IrBB4 occured only with a very modest enantioselectivity of 45% ee , thereby confirming that the hydroxy group exerts an important directing role for the incoming N -Boc-Schiff base electrophile. Figure 4: Mechanism of the aza-Henry reaction. ( a ) Proposed hydrogen-bonded ternary complex composed of a simpified derivative of iridium catalyst Λ- IrBB3 (wheat), deprotonated (nitromethyl)benzene (yellow) and N -Boc-Schiff base 5a (green) leading to the transitions state for the formation of (1 R ,2 S )- 6a . The ternary complex was built with the molecular modelling software Scigress (Fujitsu) and represented with the PyMOL Molecular Graphics System, Version 1.3 Schrödinger, LLC. ( b ) ORTEP representation with 50% probability thermal ellipsoids of a crystal structure of (1 R ,2 S )- 6g . Solvent is omitted for clarity. Full size image In conclusion, we here introduced inert octahedral 3-aminopyrazolato iridium(III) complexes as a novel class of Brønsted base catalysts and demonstrated their merit with the application to the asymmetric low-loading sulfa-Michael (down to 0.02 mol% catalyst loading) and aza-Henry reaction (down to 0.25 mol% catalyst loading) [15] . The high performance of the developed dual activation catalysts reveals the promise of octahedral metal complexes as chiral structural templates for asymmetric catalysis: their stereochemical complexity leaves large freedom in the proper arrangement of functional groups, whereas the intrinsic rigidity of the scaffold facilitates a straightforward rational design and provides entropic advantages, especially when weak interactions such as hydrogen bonds contribute to an ordered transition state. Work on expanding the scope of this novel chiral Brønsted base scaffold by tuning the basicity of the coordinated aminopyrazolato ligand is underway in our laboratory. General The synthesis and characterization of the iridium catalysts and all new substrates are provided in the Supplementary Methods . For NMR spectra, circular dichroism spectra and high-performance liquid chromatography (HPLC) traces of the iridium complexes in this article, see Supplementary Figs 1–11 . For the product analysis with HPLC on chiral stationary phase, see Supplementary Figs 12–32 . For crystallographic information, see the Supplementary Methods ; Supplementary Figs 33–35 and Supplementary Table 5 . Asymmetric sulfa-Michael addition Exemplary, a solution of 4-methylbenzenethiol ( 2a ) (49.4 mg, 0.39 mmol) in CH 2 Cl 2 (55 μl) was cooled to −78 °C and N -pyrazolylcrotonate ( 1a ) (45.1 mg, 0.33 mmol) in CH 2 Cl 2 (55 μl) was added dropwise over 1 min under an atmosphere of argon. After the mixture was stirred for 5 min, a solution of Λ- IrBB1 (0.23 mg, 0.17 μmol, 0.05 mol%) in CH 2 Cl 2 (55 μl) was added dropwise for 1 min. The resulting solution was stirred at −78 °C for additional 12 h, quenched with AcOH (1.0 ml, 0.5% v/v in n -hexane), and purified by flash chromatography on silica gel ( n -hexane/diethyl ether=50:1) to afford the product ( R )- 3a as a colourless oil (82.0 mg, 0.31 mmol, 96%). The enantiomeric excess was determined as 97% ee by HPLC using a Chiralpak OJ column (mobile phase= n -hexane/isopropanol 99:1). Experimental procedures and analytical data for this and all other sulfa-Michael additions are provided in the Supplementary Methods . For the HPLC analysis on chiral stationary phase of all sulfa-Michael addition products in this article, see Supplementary Figs 12–20 . Asymmetric aza-Henry reaction Exemplary, phenylnitromethane ( 4a ) (30.8 mg, 0.225 mmol) and Λ- IrBB3 (0.65 mg, 0.375 μmol, 0.25 mol%) were dissolved in anhydrous toluene (0.20 ml) under an atmosphere of argon and cooled to −45 °C. After being stirred for 15 min at this temperature, the Schiff base 5a (32.9 mg, 0.150 mmol), dissolved in toluene (0.10 ml), was added in one portion. The reaction was stirred for 20 h at −45 °C, then concentrated under vacuum and the pale yellow solid was purified by silica gel chromatography (CH 2 Cl 2 / n -hexane=2:5) to afford the product ( 1R , 2S )- 6a as a white solid (51.8 mg, 0.145 mmol, 97%) with 94% ee and >300:1 dr as determined by HPLC using a Chiralpak AD-H column (mobile phase= n -hexane/isopropanol 9:1). Experimental procedures and analytical data for this and all other aza-Henry reactions are provided in the Supplementary Methods . For the HPLC analysis on chiral stationary phase of all aza-Henry reaction products in this article, see Supplementary Figs 21–32 . Accession codes: The X-ray crystallographic coordinates for structures of the iridium complex Λ- IrBB1' and product ( 1R , 2S )- 6g reported in this article have been deposited at the Cambridge Crystallographic Data Centre (CCDC) under deposition numbers CCDC 1006236 and 1006234, respectively. How to cite this article: Ma, J. et al. Metal-templated chiral Brønsted base organocatalysis. Nat. Commun. 5:4531 doi: 10.1038/ncomms5531 (2014).